The collagen-binding protein ofStreptococcus mutansis involved in haemorrhagic stroke Although several risk factors for stroke have been identified, one-third remain unexplained. Here we show that infection with Streptococcus mutans expressing collagen-binding protein (CBP) is a potential risk factor for haemorrhagic stroke. Infection with serotype k S. mutans , but not a standard strain, aggravates cerebral haemorrhage in mice. Serotype k S. mutans accumulates in the damaged, but not the contralateral hemisphere, indicating an interaction of bacteria with injured blood vessels. The most important factor for high-virulence is expression of CBP, which is a common property of most serotype k strains. The detection frequency of CBP-expressing S. mutans in haemorrhagic stroke patients is significantly higher than in control subjects. Strains isolated from haemorrhagic stroke patients aggravate haemorrhage in a mouse model, indicating that they are haemorrhagic stroke-associated. Administration of recombinant CBP causes aggravation of haemorrhage. Our data suggest that CBP of S. mutans is directly involved in haemorrhagic stroke. Stroke causes 9% of all deaths worldwide and is the second most common cause of death after ischemic heart disease [1] . Strokes are primarily classified into ischemic or haemorrhagic subtypes. Several genetic and environmental risk factors for stroke have been identified. However, approximately one-third of the attributed risk remains unexplained by any detected risk factor [2] , [3] , [4] . Several types of bacterial infection including oral bacteria are reported to be associated with cardiovascular diseases [5] , [6] . As the thrombotic and thrombolytic systems are closely related to the pathogenesis of cardiovascular diseases, many studies on bacteria-induced platelet activation have been performed [7] , [8] , [9] , [10] . Most reports describe the induction of platelet activation and aggregation by various bacteria such as Staphylococcus aureus and Porphyromonas gingivalis , and their mechanisms are well investigated [7] , [8] , [9] , [10] . In contrast, there is a possibility that some bacteria may inhibit platelet aggregation. However, little is known about the clinical significance of such bacteria on cardiovascular diseases. Recently, we reported the possibility that several strains of Streptococcus mutans , a major pathogen of dental caries, may affect platelet aggregation [11] . S. mutans strains are reported to be isolated from extraoral sites, such as blood and extirpated heart valve specimens, which are presumed to be derived from the oral cavity, and dental procedures are thought to be one of the most important causes of the onset of bacteremia [12] , [13] . S. mutans are now classified into four serotypes ( c / e / f / k ), with a prevalence of more than 70% of serotype c , ∼ 20% of serotype e ,and less than 5% of serotype f and k strains in the oral cavity [14] . Serotype k was recently designated as separate from non- c / e / f serotype strains isolated from the blood of patients with bacteremia after tooth extraction [14] . Thus, S. mutans is known to be a possible pathogen for not only dental caries but also bacteremia. However, the associations between S. mutans and the other systemic diseases remain to be elucidated. There are several complicating diseases reported in patients with infective endocarditis, and 10% of these patients have been shown to be associated with intracerebral complications in Japan [15] . In addition, one of the serotype k S. mutans strains was isolated from a bacteremia patient complicated with an intracerebral vascular disorder [16] . Thus, we speculated that such S. mutans strains might be involved in the pathogenesis of intracerebral diseases. In this study, we show that infection with haemorrhagic stroke-associated S. mutans strains is a potential risk factor for cerebral haemorrhage. Our data presents a new potential risk factor for haemorrhagic stroke. Evaluation of cerebral haemorrhage in a mouse model In our experimental procedure ( Fig. 1a,b ), weak bleeding was observed in the ipsilateral hemisphere downstream of the middle cerebral artery 24 h after the induction of cerebral haemorrhage ( Fig. 1c,d ). Our mouse model reflects the haemorrhagic transformation of ischemic stroke. Administration of MT8148, the standard strain of S. mutans (serotype c strain), did not show any aggravated effects on cerebral haemorrhage in comparison to vehicle control ( Fig. 1e ). In contrast, TW871, a serotype k strain isolated from a subject with subarachnoid haemorrhage ( Supplementary Table S1 ), showed a significant exacerbation of cerebral haemorrhage ( Fig. 1e ). Similarly, the groups of mice infected with other serotype k strains, TW295 or SA53, showed significantly greater haemorrhagic areas than control or groups infected with MT8148. TW295 and SA53 caused the greatest increase in the area of cerebral haemorrhage. However, no alterations in blood pressure, heart rate or cerebral blood flow were observed after the administration of strain TW295 in a mouse stroke model ( Supplementary Tables S2, S3 ). Microscopic observations revealed obvious bleeding in TW295-administered mouse brains 3 h after the onset of cerebral haemorrhage ( Fig. 1f ). Furthermore, we investigated the effect of TW295, the most virulent strain of S. mutans , on the activation of matrix metalloproteinase (MMP)-9. Disruption of blood vessels barriers by activated MMP-9 is an important amplification pathway that causes further bleeding [17] , [18] . 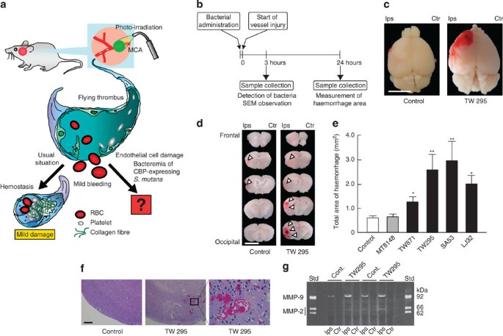Figure 1: Evaluation of the virulence of serotypek S. mutansstrains using the mouse cerebral haemorrhage model. (a) Schematic illustrations of the hypothesis and experimental procedures forS. mutans-induced aggravation of cerebral haemorrhage. (b) Schedule of experimental procedures for photochemically induced endothelial cell injury of the middle cerebral artery in mice. (c) Representative macroscopic appearance of whole mouse brain 24 h after the onset of cerebral haemorrhage administered phosphate buffered saline (PBS, vehicle control) or the TW295 strain ofS. mutans. Ips; ipsilateral, Ctr; contralateral hemisphere of brain, respectively. Scale bar; 5 mm. (d) Representative macroscopic appearance of slices of mouse brain administered PBS (control) or the TW295 strain ofS. mutans. Arrowheads indicate the haemorrhaged areas. Scale bar; 5 mm. (e) Size of the haemorrhage areas of the group of mice infected with various strains ofS. mutans. Each column represents mean±standard error (s.e.m.) from 10–21 independent experiments. Statistical significance was determined using Bonferroni's method after ANOVA. *P<0.05; **P<0.01 versus control. (f) Typical microscopic photographs of ipsilateral hemisphere isolated from control or TW295-administered mice 3 h after the onset of cerebral haemorrhage. Large magnification shows microvascular bleeding. Scale bar; 200 μm. (g) Activation of MMP-9 in mouse brain by gelatin gel zymography. Samples were collected 24 h after the administration of bacteria. Std; standard of MMP-9 (92 kDa) and MMP-2 (62 and 66 kDa). As shown in Figure 1g , activation of MMP-9 was specifically observed in the ipsilateral hemisphere of injured mouse brain. Administration of TW295 stimulated further activation of MMP-9 in the ipsilateral hemisphere compared with control. However, it should be noted that the administration of TW295 alone in the absence of injury to the cerebral artery did not cause any tissue damage in mice 24 h after the onset of cerebral haemorrhage (see the contralateral hemisphere in Fig. 1c,d ). These results indicate that the presence of both a vascular event and bacteremia of serotype k strains is required for aggravation of cerebral haemorrhage. Figure 1: Evaluation of the virulence of serotype k S. mutans strains using the mouse cerebral haemorrhage model. ( a ) Schematic illustrations of the hypothesis and experimental procedures for S. mutans -induced aggravation of cerebral haemorrhage. ( b ) Schedule of experimental procedures for photochemically induced endothelial cell injury of the middle cerebral artery in mice. ( c ) Representative macroscopic appearance of whole mouse brain 24 h after the onset of cerebral haemorrhage administered phosphate buffered saline (PBS, vehicle control) or the TW295 strain of S. mutans . Ips; ipsilateral, Ctr; contralateral hemisphere of brain, respectively. Scale bar; 5 mm. ( d ) Representative macroscopic appearance of slices of mouse brain administered PBS (control) or the TW295 strain of S. mutans . Arrowheads indicate the haemorrhaged areas. Scale bar; 5 mm. ( e ) Size of the haemorrhage areas of the group of mice infected with various strains of S. mutans . Each column represents mean±standard error (s.e.m.) from 10–21 independent experiments. Statistical significance was determined using Bonferroni's method after ANOVA. * P <0.05; ** P <0.01 versus control. ( f ) Typical microscopic photographs of ipsilateral hemisphere isolated from control or TW295-administered mice 3 h after the onset of cerebral haemorrhage. Large magnification shows microvascular bleeding. Scale bar; 200 μm. ( g ) Activation of MMP-9 in mouse brain by gelatin gel zymography. Samples were collected 24 h after the administration of bacteria. Std; standard of MMP-9 (92 kDa) and MMP-2 (62 and 66 kDa). Full size image Collagen-binding protein and cerebral haemorrhage We hypothesized that administered bacteria may specifically localize to damaged areas. Therefore, we attempted to detect S. mutans in damaged tissues in our cerebral haemorrhage model after the administration of bacteria. We observed accumulation of administered TW295 cells only in the ipsilateral hemisphere, but not other parts of the brain or organs ( Fig. 2a,b ). The number of bacteria localized to the whole ipsilateral hemisphere at 3 h after the onset of damage was 14,333±5,377. In addition, the presence of administrated bacteria in the vessels of damaged areas was detected by optical microscopic observation ( Fig. 2c ). Furthermore, apparent accumulation of administered TW295 in the damaged blood vessel was confirmed by ex vivo electron microscopic observation ( Fig. 2d ). Bacteria were localized to the endothelial cell-damaged and collagen fibre-denuded blood vessels in the ipsilateral hemisphere. Furthermore, obvious binding of bacteria to collagen fibres was also confirmed in the damaged vessels ( Fig. 2e ). These results suggest that the administered bacteria specifically interacted with damaged vessels in vivo , especially via denuded collagen fibres. 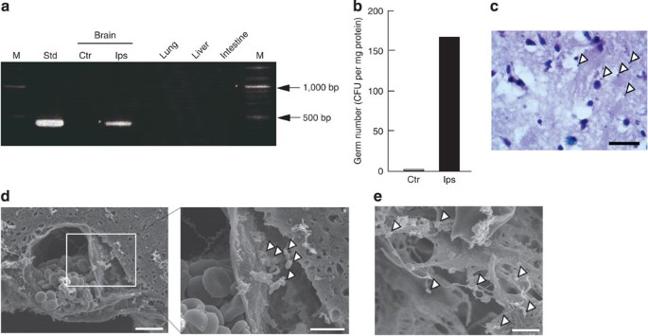Figure 2: Accumulation of administered bacteria in damaged ipsilateral area of mouse brain. (a) Detection of the infected bacterial cells in various kinds of organs by PCR. M; Molecular marker (100-bp ladder, bold bands are 1,000 bp and 500 bp, respectively), Std; Positive control of the genomic DNA extracted from TW295. Ips; ipsilateral, Ctr; contralateral hemisphere of brain, respectively. (b) Recovered isolation of administered bacteria in damaged or non-damaged area. Samples isolated from damaged or non-damaged area in brains were plated onto culture dish for collecting ofS. mutans. Recovered isolation numbers of bacteria are expressed as CFU per mg protein. Each column represents mean value from three independent animals. (c) Detection of accumulated bacteria in damaged brain areas by Gram-stain. White arrowheads indicate the accumulated bacteria. Scale bar; 25 μm. (d) Representative appearance of the interaction of the injured blood vessel and infected bacterial cells observed byin vivoSEM. Scale bar; 10 μm. The right photo shows high magnification. White arrowheads show the accumulated bacteria leaked outside of the vessel at the injured site. Scale bar; 5 μm. (e) Interaction of bacteria and collagen fibres around the vessels in a damaged hemisphere byin vivoSEM. White arrowheads indicate bacteria interacting with collagen fibres. Scale bar; 2 μm. Figure 2: Accumulation of administered bacteria in damaged ipsilateral area of mouse brain. ( a ) Detection of the infected bacterial cells in various kinds of organs by PCR. M; Molecular marker (100-bp ladder, bold bands are 1,000 bp and 500 bp, respectively), Std; Positive control of the genomic DNA extracted from TW295. Ips; ipsilateral, Ctr; contralateral hemisphere of brain, respectively. ( b ) Recovered isolation of administered bacteria in damaged or non-damaged area. Samples isolated from damaged or non-damaged area in brains were plated onto culture dish for collecting of S. mutans . Recovered isolation numbers of bacteria are expressed as CFU per mg protein. Each column represents mean value from three independent animals. ( c ) Detection of accumulated bacteria in damaged brain areas by Gram-stain. White arrowheads indicate the accumulated bacteria. Scale bar; 25 μm. ( d ) Representative appearance of the interaction of the injured blood vessel and infected bacterial cells observed by in vivo SEM. Scale bar; 10 μm. The right photo shows high magnification. White arrowheads show the accumulated bacteria leaked outside of the vessel at the injured site. Scale bar; 5 μm. ( e ) Interaction of bacteria and collagen fibres around the vessels in a damaged hemisphere by in vivo SEM. White arrowheads indicate bacteria interacting with collagen fibres. Scale bar; 2 μm. Full size image Therefore, we focused on a direct interaction between serotype k S. mutans and collagen fibres. It is well known that denuded collagen fibres exist on the surface of damaged vessels after the rupture of endothelial cells, and the interaction between collagen fibres and platelets is important for the initiation of platelet aggregation. Recently, a cell-surface 120-kDa collagen-binding adhesin (Cnm) was identified in S. mutans , and its coding gene ( cnm ) was cloned and sequenced [19] . In our previous study, the distribution of cnm in S. mutans clinical strains was shown to be ∼ 10%, and its distribution was predominant in serotype k or f strains [20] , [21] . Interestingly, all of the highly virulent strains (TW871, TW295, SA53 and LJ32, see Fig. 1e ) observed in cerebral haemorrhage cases have this surface collagen-binding protein (CBP) ( Supplementary Table S1 ). In fact, collagen-binding activity of the highly virulent strains was dramatically higher than that of MT8148 in vitro ( Fig. 3a ). In addition, platelet aggregation was decreased in vitro after treatment with the highly virulent strains in comparison to MT8148 ( Fig. 3b ). Therefore, we generated a mutant strain with a CBP expression defect (TW295CND, Supplementary Table S1 ) from the TW295 strain [21] . This strain completely lost the ability to bind to collagen ( Fig. 3a ). The suppression of platelet aggregation observed with TW295 was completely ameliorated with TW295CND ( Fig. 3b ). These results clearly indicate that CBP is necessary for the collagen-binding activity and inhibition of platelet aggregation observed with the TW295 strain. Next, we administered the TW295CND strain to mice in our cerebral haemorrhage model. 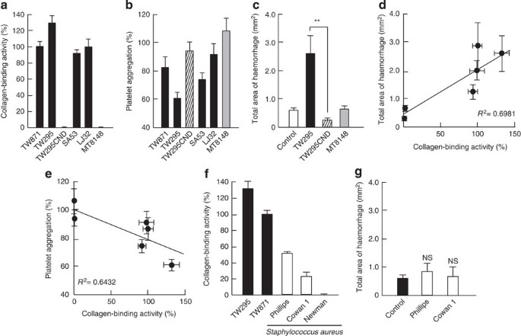Figure 3: Relationship between collagen-binding activity and cerebral haemorrhage. (a) Collagen-binding activity of various strains ofS. mutans. The activity was evaluated under fixed conditions of 2 mg of Type I collagen and 1×1010bacterial cells. The results for each strain are expressed as a percentage of TW871 (defined as 100%). Each column represents mean±standard deviation (s.d.) from three independent experiments. (b) Platelet aggregation activity of various strains ofS. mutans. The assays were performed using whole blood obtained from mice with an aggregometer under fixed conditions of 4 μg of Type I collagen and 1×107bacterial cells. The results for each strain are expressed as a percentage based on that with collagen but no bacterial cells as 100%. Each column represents mean±s.d. from 3–5 independent experiments. (c) Size of the haemorrhagic areas of mice infected with TW295, TW295CND (the strain generated from TW295), or MT8148. Each column represents mean±s.e.m. from 11–16 independent experiments Statistical significance was determined using Bonferroni's method after ANOVA. **P<0.01 versus TW295. (d) Correlation between collagen-binding activity and total area of haemorrhage (regression analysis;R2=0.6981). Each point represents mean±s.e.m. from the data of each treatment. (e) Correlation between collagen-binding activity and collagen-induced platelet aggregation (regression analysis;R2=0.6432). Each point represents mean±s.e.m. from the data of each treatment. (f) Collagen-binding activity of various strains ofS.aureus. Phillips and Cowan 1 are reported to have high collagen-binding activity in variousS. aureusstrains. The activity was evaluated under fixed conditions of 2 mg of Type I collagen and 1×1010bacterial cells. The results for each strain are expressed as a percentage of TW871 activity as 100%. Each column represents mean±s.d. from 3–5 independent experiments. (g) Size of the haemorrhagic areas of mice infected with the two strains ofS. aureusin a mouse stroke model. Each column represents mean±s.e.m. from 6–7 independent experiments. NS; no statistical significance versus control (Bonferroni's method after ANOVA). As shown in Figure 3c , a drastic reduction in cerebral haemorrhage area was observed in mice administered TW295CND in comparison to those administered TW295. A good correlation between collagen-binding activity and haemorrhage area ( Fig. 3d ) and inhibition of platelet aggregation ( Fig. 3e ) was observed. These results indicate that CBP in serotype k S. mutans is the main cause of its high virulence in cerebral haemorrhage. Figure 3: Relationship between collagen-binding activity and cerebral haemorrhage. ( a ) Collagen-binding activity of various strains of S. mutans . The activity was evaluated under fixed conditions of 2 mg of Type I collagen and 1×10 10 bacterial cells. The results for each strain are expressed as a percentage of TW871 (defined as 100%). Each column represents mean±standard deviation (s.d.) from three independent experiments. ( b ) Platelet aggregation activity of various strains of S. mutans . The assays were performed using whole blood obtained from mice with an aggregometer under fixed conditions of 4 μg of Type I collagen and 1×10 7 bacterial cells. The results for each strain are expressed as a percentage based on that with collagen but no bacterial cells as 100%. Each column represents mean±s.d. from 3–5 independent experiments. ( c ) Size of the haemorrhagic areas of mice infected with TW295, TW295CND (the strain generated from TW295), or MT8148. Each column represents mean±s.e.m. from 11–16 independent experiments Statistical significance was determined using Bonferroni's method after ANOVA. ** P <0.01 versus TW295. ( d ) Correlation between collagen-binding activity and total area of haemorrhage (regression analysis; R 2 =0.6981). Each point represents mean±s.e.m. from the data of each treatment. ( e ) Correlation between collagen-binding activity and collagen-induced platelet aggregation (regression analysis; R 2 =0.6432). Each point represents mean±s.e.m. from the data of each treatment. ( f ) Collagen-binding activity of various strains of S . aureus . Phillips and Cowan 1 are reported to have high collagen-binding activity in various S. aureus strains. The activity was evaluated under fixed conditions of 2 mg of Type I collagen and 1×10 10 bacterial cells. The results for each strain are expressed as a percentage of TW871 activity as 100%. Each column represents mean±s.d. from 3–5 independent experiments. ( g ) Size of the haemorrhagic areas of mice infected with the two strains of S. aureus in a mouse stroke model. Each column represents mean±s.e.m. from 6–7 independent experiments. NS; no statistical significance versus control (Bonferroni's method after ANOVA). Full size image It was reported that several strains of S. aureus also expressed CBP [22] , [23] . We, therefore, investigated the effect of such S. aureus strains on collagen-binding activity and aggravation of haemorrhage. As shown in Fig. 3f , the collagen-binding activity of S. aureus strains was much lower than that of TW295-type S. mutans . Aggravation of haemorrhage by S. aureus was not observed ( Fig. 3g ). These results may indicate that not only the bacterial characteristics, but also the characteristics of CBP differ between S. mutans and S. aureus . Inhibition of platelet aggregation by serotype k strains Platelet aggregation is the most important step to hemostasis after vascular damage. Therefore, we investigated the effect of various serotypes of S. mutans on collagen-induced platelet aggregation. MT8148, the standard strain of S. mutans , did not show any inhibitory effects on platelet aggregation in whole blood in comparison to vehicle control ( Supplementary Fig. S1a ). In contrast, TW871, a serotype k strain, showed a significant inhibition of collagen-induced platelet aggregation, when 10 7 cells were added to whole blood. We also investigated the effects of 58 other clinically isolated S. mutans strains on collagen-induced platelet aggregation. The aggregation rates of serotype k strains were significantly lower than those of other serotypes ( Supplementary Fig. S1b ). Among them, the TW295 strain showed the most potent inhibition of collagen-induced platelet aggregation. Interestingly, platelet aggregation rates of blood-isolated strains were shown to be significantly lower than those of orally isolated strains ( Supplementary Fig. S1c ). Further results were obtained when TW871 was added to the platelet aggregation system using platelet-rich plasma (PRP, Supplementary Fig. S2a,b ). Maximum aggregation, induced by the addition of collagen, was dramatically decreased by the addition of TW871, but not MT8148, a standard strain. An increase in the lag-time to the onset of aggregation was also observed ( Supplementary Fig. S2c ). In addition, bleeding time in mice showed a tendency to be prolonged after TW295 administration (control; 170±10.0 s. versus TW295; 180±14.5 s., n =6, mean±s.e.m.). However, arachidonic acid-induced platelet aggregation was not inhibited by the administration of TW295 ( Supplementary Fig. S2d ). Therefore, we hypothesized that TW295 might be intercepting collagen, resulting in the inhibition of platelet activation. 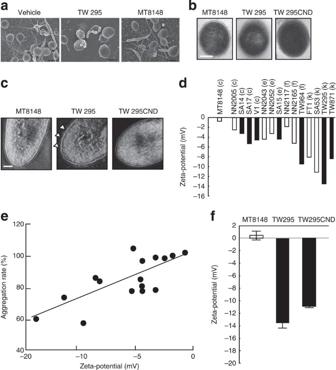Figure 4: Variation of bacterial cell surface conditions and collagen-induced platelet aggregation. (a) Representative appearance ofS. mutansstrains and platelet reactions to collagen observed by SEM. After the reaction with collagen, the platelet fraction was collected and observed by SEM. Scale bar; 2 μm. (b) TEM observation of bacterial surfaces. Scale bar; 0.2 μm. (c) Three-dimensional reconstructed images of bacterial surface of MT8148, TW295 and TW295CND. Opaque with a vague appearance of the peptidoglycan layer of TW295 is indicated with arrowheads. Scale bar; 0.1 μm. (d) Zeta-potential values ofS. mutansstrains. Zeta-potential values of various strains were measured and expressed in mV. Open columns represent oral isolates and closed columns blood isolates. Each column represents the mean value from 3–5 independent experiments. (e) Correlation between platelet aggregation and zeta-potential value (regression analysis;R=0.740,P=0.0011). Each point represents a mean value from each bacterial strain. (f) Comparison of zeta potential values on MT8148, TW295, and TW295CND. Each column represents mean±s.e.m. from 3–5 independent experiments. As shown in the scanning electron microscopic (SEM) images in Figure 4a , interactions between platelets and collagen that result in platelet activation were observed when the platelet fraction was collected after stimulation with collagen ( Fig. 4a ). Morphological changes associated with platelet activation, such as pseudopodia and platelet adhesion, were observed in the vehicle control group. Addition of MT8148 did not show any effects on the interaction of platelets and collagen versus control ( Fig. 4a , MT8148). In contrast, the addition of TW295 showed obvious suppression of the interaction between platelets and collagen, resulting in the inhibition of platelet activation ( Fig. 4a , TW295). These results clearly indicate that the binding of collagen by TW295 leads to inhibition of the interaction between platelets and collagen, resulting in the inhibition of aggregation. Figure 4: Variation of bacterial cell surface conditions and collagen-induced platelet aggregation. ( a ) Representative appearance of S. mutans strains and platelet reactions to collagen observed by SEM. After the reaction with collagen, the platelet fraction was collected and observed by SEM. Scale bar; 2 μm. ( b ) TEM observation of bacterial surfaces. Scale bar; 0.2 μm. ( c ) Three-dimensional reconstructed images of bacterial surface of MT8148, TW295 and TW295CND. Opaque with a vague appearance of the peptidoglycan layer of TW295 is indicated with arrowheads. Scale bar; 0.1 μm. ( d ) Zeta-potential values of S. mutans strains. Zeta-potential values of various strains were measured and expressed in mV. Open columns represent oral isolates and closed columns blood isolates. Each column represents the mean value from 3–5 independent experiments. ( e ) Correlation between platelet aggregation and zeta-potential value (regression analysis; R =0.740, P =0.0011). Each point represents a mean value from each bacterial strain. ( f ) Comparison of zeta potential values on MT8148, TW295, and TW295CND. Each column represents mean±s.e.m. from 3–5 independent experiments. Full size image Furthermore, we investigated the cell surface differences between MT8148 and TW295 using electron microscopy. Transmission electron microscopic observation (TEM, Fig. 4b ) showed differences in cell surface between MT8148 and the serotype k strain TW295. However, the appearance of bacterial membranes by TEM of ultrathin sections can sometimes vary with observational direction. In addition, it is necessary to consider section thickness during ultrastructural observations. Therefore, we compared the bacterial membrane using three-dimensional images re-constructed by computed tomography (CT) of TEM. As shown in Fig. 4c , the peptidoglycan layer of MT8148 appeared as a clear and smooth layer in the three-dimensional TEM image. In contrast, the peptidoglycan layer of TW295 was opaque with a vague appearance. These results indicate that the differences in the bacterial surface, including the peptidoglycan layer, may affect the binding of bacteria to collagen fibres. The surface ionic charge of platelets is one of the important factors leading to interaction with exposed collagen fibres on injured blood vessels. The anionic character of the platelet surface leads to interactions with the cationic charges of collagen [24] , [25] , [26] . Therefore, we determined the ionic charge of the bacterial surface, because it may affect bacterial interactions with collagen. The mean values for zeta-potential, as an index of cell surface ionic charge, of MT8148 cells dissolved in saline was −0.75 mV, indicating an almost nonionic character ( Fig. 4d ). The zeta-potential values of serotype k strains such as TW295 and TW871 were much lower than that of MT8148, indicating that the cell surface of serotype k strains was anionic. A regression analysis between the zeta-potential value and the platelet aggregation rate showed a significant positive correlation ( Fig. 4e ). Thus, a vague peptidoglycan layer on the bacterial surface may affect the surface ionic charge, altering the binding strength between bacteria and collagen fibres. In contrast, the zeta potential value and cell surface layer of the CBP-defective strain, TW295CND, was slightly, but not markedly, changed versus MT8148 ( Fig. 4f ), Thus, CBP itself may not be the only determinant of cell surface conditions such as zeta potential and peptidoglycan structure. Strains isolated from stroke patients caused haemorrhage To further support our hypothesis that the infection of CBP-expressing S. mutans is a potential risk factor for haemorrhagic stroke, we compared the frequency of cnm -expressing (CBP-expressing) S. mutans in oral samples between cerebral haemorrhage patients and age-matched non-stroke healthy subjects. S. mutans was isolated from 41 out of 74 patients. Among them, 20 patients were infected with cnm -expressing S. mutans (20/41, 48.8%, Table 1 ). The frequency of cnm -expressing TW295-type S. mutans strains in cerebral haemorrhage patients was significantly higher than that in control subjects (control; 3/20, 15.0%, Table 1 , Odds ratio 5.40). In addition, we compared the frequency of cnm -expressing S. mutans strains between cerebral haemorrhage and ischemic (non-haemorrhagic) stroke patients. The frequency of cnm -expressing S. mutans strains was significantly higher in cerebral haemorrhage than ischemic stroke patients ( Supplementary Table S4 ). These results suggested that infection of CBP ( cnm )-expressing S. mutans is a potential risk factor for haemorrhagic stroke. In addition, we tested the virulence of CBP-expressing S. mutans strains isolated from patients. We tested two CBP-expressing S. mutans strains from stroke patients (SMH2 and SMH4) in a mouse haemorrhagic stroke model, because they showed both strong collagen-binding activity and inhibition of collagen-induced platelet aggregation ( Supplementary Fig. S3a,b ). A dramatic aggravation of cerebral haemorrhage was observed in mice administered with the two isolated cnm -expressing S. mutans strains in comparison to control ( Fig. 5a,b,c ). These results clearly indicate that infection of CBP-expressing S. mutans from cerebral haemorrhage patients is a risk factor for haemorrhagic stroke. Table 1 Frequency of cnm -expressing S. mutans infection in cerebral haemorrhage patients and control subjects. 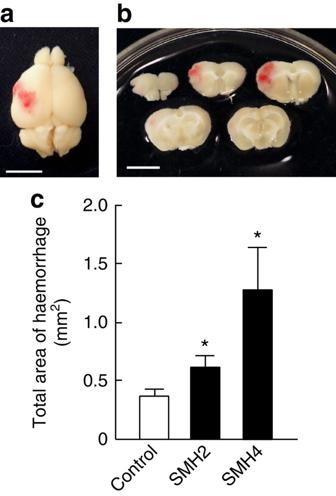Figure 5: Effect of CBP-expressingS. mutansisolated from stroke patients on cerebral haemorrhage. (a) Representative macroscopic appearance of whole mouse brain 24 h after the onset of cerebral haemorrhage administered SMH4 isolated from a haemorrhagic stroke patient. Scale bar; 5 mm. (b) Representative macroscopic appearance of mouse brain slices administered SMH4. Scale bar; 5 mm. (c) Size of the haemorrhage areas from the group of mice infected with CBP-expressingS. mutans(SMH2 and SMH4) isolated from stroke patients. Each column represents mean±s.e.m. from 11–16 independent experiments. Statistical significance was determined using Bonferroni's method after ANOVA. *P<0.05 versus control. Full size table Figure 5: Effect of CBP-expressing S. mutans isolated from stroke patients on cerebral haemorrhage. ( a ) Representative macroscopic appearance of whole mouse brain 24 h after the onset of cerebral haemorrhage administered SMH4 isolated from a haemorrhagic stroke patient. Scale bar; 5 mm. ( b ) Representative macroscopic appearance of mouse brain slices administered SMH4. Scale bar; 5 mm. ( c ) Size of the haemorrhage areas from the group of mice infected with CBP-expressing S. mutans (SMH2 and SMH4) isolated from stroke patients. Each column represents mean±s.e.m. from 11–16 independent experiments. Statistical significance was determined using Bonferroni's method after ANOVA. * P <0.05 versus control. Full size image Analysis of stroke prone spontaneous hypertensive rat model To test whether TW295-type S. mutans also aggravates cerebral haemorrhage in other stroke model and animal species, we used the stroke prone spontaneous hypertensive (SHRSP) rat model. As the SHRSP rat exhibits spontaneous stroke induced by hypertension, we exposed SHRSP rats to TW295 ( Supplementary Fig. S4 ). 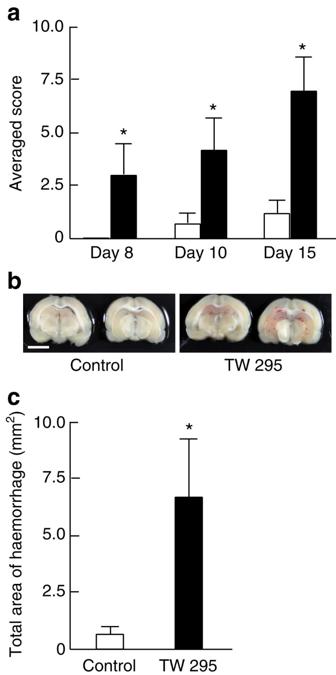Figure 6: Effect of CBP-expressingS. mutanson SHRSP rats. (a) Alteration of neurological deficits on TW295-administered or vehicle-administered SHRSP rats. The neurological deficit score of each animal was evaluated and scored. Open columns represent vehicle-administered control and closed columns represent TW295 administered groups. Each column represents mean±s.e.m. from 8–10 independent experiments. Statistical significance was determined using Student'st-test. *P<0.05 versus control. (b) Representative macroscopic appearance of SHRSP rat brain slices administered TW295 (TW295) or vehicle (Control). Scale bar; 5 mm. (c) Total size of the haemorrhage areas of the group of SHRSP rats injected with TW295 or vehicle (control). Each column represents mean±s.e.m. from 8–10 independent experiments. Statistical significance was determined using Student'st-test. *P<0.05 versus control. As shown in Figure 6 , the group administered TW295 showed obvious neurological deficits, such as forelimb and hindlimb flexion, forelimb motor function, postural reaction, and abnormal posture in comparison to vehicle-administered control SHRSP rats ( Fig. 6a and Supplementary Movies 1 , 2 ). Increased haemorrhage in the whole brain of TW295-administered SHRSP rats was clearly observed in comparison to that of vehicle-administered control SHRSP rats ( Fig. 6b,c ). These results clearly indicate that aggravation of cerebral haemorrhage induced by TW295 occurs in multiple stroke models, and may be a common mechanism between various animal species, including human. Figure 6: Effect of CBP-expressing S. mutans on SHRSP rats. ( a ) Alteration of neurological deficits on TW295-administered or vehicle-administered SHRSP rats. The neurological deficit score of each animal was evaluated and scored. Open columns represent vehicle-administered control and closed columns represent TW295 administered groups. Each column represents mean±s.e.m. from 8–10 independent experiments. Statistical significance was determined using Student's t -test. * P <0.05 versus control. ( b ) Representative macroscopic appearance of SHRSP rat brain slices administered TW295 (TW295) or vehicle (Control). Scale bar; 5 mm. ( c ) Total size of the haemorrhage areas of the group of SHRSP rats injected with TW295 or vehicle (control). Each column represents mean±s.e.m. from 8–10 independent experiments. Statistical significance was determined using Student's t -test. * P <0.05 versus control. Full size image Aggravation of haemorrhage by recombinant Cnm protein As CBP-expressing S. mutans causes the aggravation of cerebral haemorrhage, we hypothesized that CBP itself might be able to cause haemorrhage. To clarify the role of CBP in the aggravation of haemorrhage, we produced recombinant Cnm protein. Pre-application of 100 μg recombinant Cnm protein completely inhibited TW295 binding to the collagen layer, indicating that recombinant Cnm protein functionally binds to the collagen layer ( Supplementary Fig. S5 ). We then administered recombinant Cnm protein in a mouse stroke model. 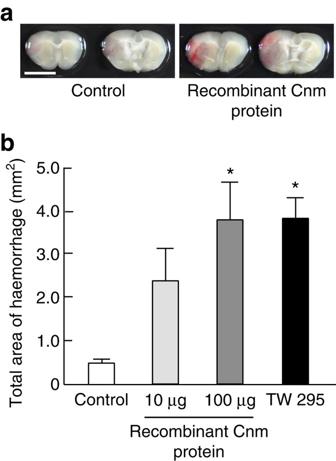Figure 7: Effect of recombinant Cnm protein administration in a mouse cerebral haemorrhage model. (a) Macroscopic appearance of representative mouse brain slices administered recombinant Cnm protein or vehicle (Control). Scale bar; 5 mm. (b) Total size of the haemorrhage areas of the mice administered recombinant Cnm protein (10 and 100 μg per animal), TW295 bacterial cells (TW295), or vehicle (Control). Each column represents mean±s.e.m. from 10–12 independent experiments. Statistical significance was determined using Bonferroni's method after ANOVA. *P<0.05 versus control. As shown in Figure 7 , administration of recombinant Cnm protein dose-dependently aggravated cerebral haemorrhage. A dosage of 100 μg of recombinant Cnm protein showed a similar degree of haemorrhagic aggravation compared with TW295 administration ( Fig. 7b ). These results indicate that CBP itself can aggravate cerebral haemorrhage. Figure 7: Effect of recombinant Cnm protein administration in a mouse cerebral haemorrhage model. ( a ) Macroscopic appearance of representative mouse brain slices administered recombinant Cnm protein or vehicle (Control). Scale bar; 5 mm. ( b ) Total size of the haemorrhage areas of the mice administered recombinant Cnm protein (10 and 100 μg per animal), TW295 bacterial cells (TW295), or vehicle (Control). Each column represents mean±s.e.m. from 10–12 independent experiments. Statistical significance was determined using Bonferroni's method after ANOVA. * P <0.05 versus control. Full size image This is the first study showing that infection with CBP-expressing S. mutans is a potential risk factor for haemorrhagic stroke. Bacteria-related aggravation of cerebral haemorrhage was demonstrated in mice infected with serotype k S. mutans strains. In addition, administered bacteria were identified in the ipsilateral but not the contralateral hemisphere, indicating that the interaction of serotype k S. mutans with damaged blood vessels is a crucial event in the development of the cerebral haemorrhage. Aggravation of cerebral haemorrhage induced by serotype k S. mutans strains may be a common effect between various animal species, including humans, because the aggravation by TW295 was also observed in the SHRSP rat stroke model. The serotype k S. mutans strains exhibited common cell surface protein expression patterns, including the expression of CBP that could be important for the aggravation of cerebral haemorrhage. Our hypothesis that CBP of serotype k S. mutans is necessary for cerebral haemorrhage is supported by our result that the CBP-defective mutant strain, TW295CND, showed no aggravation of cerebral haemorrhage. The highly virulent strains, TW295, TW871, SA53 and LJ32 (although LJ32 is not serotype k ), commonly possessed strong collagen-binding properties because of their cell surface CBP expression. As collagen-induced, but not arachidonic acid-induced, platelet aggregation was inhibited by the treatment with CBP-expressing S. mutans , interaction between collagen and CBP-expressing S. mutans may be important. We speculate that strains with strong collagen-binding properties accumulate on exposed collagen layers after the rupture of endothelial cells. With no bacteria present, platelets bind to the exposed collagen layer when the endothelial cells are damaged or ruptured. In the presence of CBP-expressing S. mutans , however, these bacteria bind to the exposed collagen layer instead of platelets, resulting in damaged areas remaining unsealed. Thus, continued bleeding may occur. In fact, we observed that a comparatively large amount of the collagen layer was exposed in the damaged hemisphere in our mouse haemorrhagic stroke model ( Supplementary Fig. S6a ) and that many bacteria accumulated in the area ( Supplementary Fig. S6b ). The accumulation of such high-virulence strains may then activate MMP-9, recruit leukocytes, and inhibit further collagen-induced platelet aggregation, resulting in further bleeding. Thus, the strains with CBP should be regarded as highly virulent strains for cerebral haemorrhage. In fact, ex vivo SEM images of blood vessels in the ipsilateral side of damaged mouse brain showed administered bacteria with no associated platelet aggregations. In addition, a slight increase in the accumulation of inflammatory cells was also observed in the ipsilateral hemisphere ( Supplementary Fig. S7 ), indicating the limited involvement of infiltrating leukocytes on the activation of MMP-9 in bacteria-administered mouse brains. Bacterial cell surface conditions, including the peptidoglycan layer and/or ionic charge, may also affect the binding of bacteria with collagen fibres. In general, collagen is cationic in physiological situations and, therefore, bacterial surface ionic character might be important for interaction with exposed collagen fibres. As the values of zeta-potential and the collagen-induced platelet aggregation rates were positively correlated, strains with low zeta-potential values (anionic) might also be classified as highly virulent strains. Taken together, we speculate that the S. mutans strains with CBP possess a high affinity to the exposed collagen fibres and that a strongly anionic cell-surface leads to further increased affinity for cationic collagen fibres. Therefore, synergism between the presence of CBP and anionic cell surface conditions may cause strong binding to collagen fibres, resulting in the accumulation of highly virulent bacteria in collagen-denuded blood vessels. We propose a mechanism of haemorrhagic aggravation of stroke in which accumulated highly virulent bacteria bind to the exposed collagen layer after endothelial cell injury, resulting in the inhibition of collagen-induced platelet aggregation in injured blood vessels. Consequently, the accumulation of bacteria leads to the activation of MMP-9, resulting in an acceleration of bleeding and haemorrhagic stroke ( Supplementary Fig. S8 ). The estimated rate of oral cavity infection by S. mutans with CBP in healthy subjects is 8–10% (refs [20] , [27] 20,27). Thus, only a limited number of strains are possible risk factors for the aggravation of cerebral haemorrhage caused by S. mutans -induced bacteremia. Therapeutic interventions for cerebral haemorrhage are limited after the onset of disease, and prevention is considered the most important approach [28] . Therefore, it may be important to identify subjects with highly virulent strains of S. mutans at risk for cerebral haemorrhage. In fact, we isolated cnm -expressing highly virulent TW295-type- S. mutans strains from haemorrhagic stroke patients with extremely high frequencies (48.8% of S. mutans -positive patients, and 27.0% of all patients) compared with age-matched non-stroke control subjects (15.0% of S. mutans positive patients, and 8.5% of all control subjects) or ischemic stroke patients (22.2% of S. mutans -positive patients, and 11.1% of all ischemic stroke patients). Thus, about 30% of cerebral haemorrhage patients have these dangerous strains. These results indicate that the bacteremia of highly virulent TW295-type S. mutans may be an important risk factor for haemorrhagic stroke in many clinical cases. In addition, several S. mutans strains with CBP isolated from stroke patients caused aggravation of cerebral haemorrhage in a mouse haemorrhagic stroke model, indicating the potential involvement of highly virulent S. mutans in occurrences of haemorrhagic stroke. Further large-scale clinical screening investigations about the relationship between the infection of highly virulent S. mutans and the occurrence of haemorrhagic stroke are required. To our surprise, administration of recombinant Cnm protein itself aggravated cerebral haemorrhage in a mouse haemorrhagic stroke model. These results clearly indicate that CBP itself is capable of causing an aggravation of cerebral haemorrhage. At the same time, it may suggest that we must be aware of the release of CBP from bacteria into circulation after destroying TW295-type S. mutans during transitory bacteremia. Free CBP may itself be a risk factor for haemorrhagic stroke. In conclusion, infection with highly virulent haemorrhagic stroke-inducible S. mutans is a potential risk factor for haemorrhagic stroke. The important identified virulence factors for cerebral haemorrhage are the presence of CBP and the anionic cell surface conditions, which are common properties of most serotype k clinical isolates. Ethics of animal experiments and human subjects All animal experiments in the present study conformed to the Guide for the Care and Use of Laboratory Animals published by the United States National Institutes of Health, and were approved by the institutional animal care and use committees of Osaka University Graduate School of Dentistry and Hamamatsu University School of Medicine. Study protocols using human samples were approved by the Ethics Committee of Osaka University Graduate School of Dentistry, Seirei Hamamatsu General Hospital, and Suita Municipal Hospital. All subjects were informed of the protocols and gave written consent before their participation in this study. Cerebral haemorrhage patients were strictly selected by neurosurgery experts using MRI and other diagnostic criteria. We also selected ischemic stroke (including atherosclerotic stroke) patients who were diagnosed with ischemic stroke without any haemorrhage. Oral samples were collected from patients in multiple institutes and hospitals. Age-matched non-stroke subjects who did not have a history of any other diseases such as stroke, heart failure, diabetes mellitus, rheumatoid arthritis, liver disease, kidney disease, gastrointestinal disease, hypertension or anemia were defined as control subjects. Bacterial strains and culture conditions Supplementary Table S1 shows the major S. mutans strains used in this study [14] , [16] , [20] , [21] , [29] . In addition, 58 clinical S. mutans strains (blood isolates; n =13; oral isolates; n =45) were selected from our laboratory stock in this study [30] . All strains were grown in brain heart infusion broth (Difco) and erythromycin was added for selection of mutant strains. S. aureus strains that have collagen-binding activity (Phillips, Cowan 1, and Newman) were also cultured in brain heart infusion broth [22] , [23] . Collagen-binding assay The collagen-binding properties were evaluated according to the method described by Waterhouse and Russell [31] , with some modifications [27] . The activity was evaluated under fixed conditions of 2 mg of Type I collagen and 1×10 10 bacterial cells. The results for each strain are expressed as a percentage compared with TW871 binding, which was defined as 100%. Platelet aggregation assay The platelet aggregation assay was carried out using mouse whole blood by an impedance method with an aggregometer (Whole-blood aggregometer C540, Baxter). Briefly, whole blood was taken from mice (ICR, male, 8-weeks-old, CLEA), and mixtures of varied amounts of bacterial cells (10 3 –10 7 colony forming unit, CFU) and whole blood were incubated at 37 °C for 5 min, followed by the addition of collagen (native collagen fibrils (type I), Chrono-log). Aggregation rates of each strain were calculated by impedance (Ω) values with or without the addition of bacterial cells, and were expressed as a percent of vehicle. In addition to the whole blood aggregation, we performed a platelet aggregation assay using human PRP. Human PRP was prepared from healthy volunteers and the standard S. mutans strain, MT8148, or TW871 (final concentration; 10 7 cells ml −1 ) was added. Collagen (4 μg) was added 5 min after the incubation with MT8148 or TW871, and the maximum impedance value during the 20-min. observation period was measured using an aggregometer. Maximum platelet aggregation rates and the prolongation of lag-time until the start of aggregation were evaluated using PRP. Evaluation of bacterial surface charge Bacterial surface charge was evaluated as zeta-potential values using a zeta-potential analyzer (ELSZ-2, Otsuka Electronics), which automatically calculated zeta-potential from the electrophoresis mobility using the Smoluchowski equation. Overnight-cultured bacterial cells were washed and adjusted using PBS to 10 7 CFU and were applied to the analyzer, which measured the zeta-potential of the cells at five standard points automatically. Results were expressed as mean values. Mouse cerebral haemorrhage model Endothelial injury in middle cerebral artery of mice was induced using a photochemical method with some modifications [17] , [32] ( Fig. 1a,b ). Bacterial suspensions (10 7 cells per body) in PBS were intravenously administered through the jugular vein, followed by the administration of rose bengal under photo-irradiation with a xenon lamp equipped with a heat-absorbing filter (0.04 W cm −2 , wavelength 540 nm, Hamamatsu Photonics) for 10 min using a 1.5-mm diameter optic fibre mounted on a micromanipulator. Twenty-four hours after the bacterial infection, mice were sacrificed and the brains were removed. The total haemorrhage areas from all brain sections were calculated by computer analysis and expressed in mm 2 according to the method [17] , [32] (DP controller, model DP70, Olympus). Activation of matrix metalloprotease-9 Gelatin gel zymography was performed according to the method of Gursoy-Ozdemir et al . with some modifications [18] . Briefly, tissue samples collected 24 h after the administration of bacteria or vehicle were homogenized in 50 mM Tris–HCl, 150 m M NaCl, 1% Nonidet P-40, 0.1% SDS and 0.1% deoxycholic acid, pH 7.4 buffer solution including protease inhibitors. Then, samples were separated by electrophoresis using a gelatin zymography-electrophoresis kit (Cosmo Bio). Ex vivo electron microscopic observation Brain tissues were removed from mice 3 h after the induction of cerebral haemorrhage for electron microscopic observations in haemorrhagic areas. Briefly, the haemorrhagic cerebrum was fixed with 2% glutaraldehyde. Then the cerebrum was cut and removed including a part of the obstacle, and were fixed again with 1% osmium tetra-oxide and dehydrated with an ethanol series. The samples were frozen and fractured into two to four pieces by a freeze fracture device filled with liquid nitrogen. The fracture surface was perpendicular to the cerebral surface, and included the haemorrhage. The fractured samples were dried with t- butyl alcohol using freeze drying equipment and adhered to the sample stage using conductive paste with the section at the top, and were then coated with osmium as conductive processing. The completed specimens were observed by SEM. Three-dimensional computed tomography of bacteria The bacterial membranes were compared using three-dimensional re-constructed images made by computed tomography (CT) of TEM (JEM 1220: JEOL). TEM images of the bacteria were taken at 150,000 magnification at every degree from a tilted range of −60° to +60°. The CT images of the three-dimensional reconstruction were produced with Radon transform software. These CT images can be displayed in an arbitrary direction. Detection of bacteria in tissue samples Detection of the infected bacteria in several organs was carried out by PCR as follows. Whole DNA was extracted from extirpated tissue, such as injured or uninjured brain hemispheres, lung, liver and intestine. PCR was carried out using S. mutans -specific sets of primers described previously [14] , [20] , [27] ( Supplementary Table S5 ). The limit of detection for bacteria was 5–50 cells in each specimen. To confirm that viable strains were in the tissue, each extirpated tissue was squeezed in sterile PBS, and the original as well as the diluted liquid were streaked on Mitis-Salivarius agar (Difco) plates containing bacitracin (100 units per ml; Sigma-Aldrich), which are the selected culture agar plates for S. mutans . Stroke model in stroke prone spontaneous hypertensive rats Male SHRSP rats (12-weeks-old, SLC) were housed in a climate-controlled (temperature 22–24 °C, humidity 40–60%) light-regulated room with a 12-h light: 12-h dark cycle. All rats consumed the SP diet (Funahashi). Free access to rat chow and 0.5% saline solution was maintained throughout the experiment. The rats were divided into two groups, a TW295-administered and a vehicle-administered control group. TW295 was administered intravenously through the tail vein at day 1, 3, 8 and 10 ( Supplementary Fig. S4a ). Non-invasive blood pressure was measured by tail cuff just before and one day after first administration of TW295 or vehicle. Body weight measurement and neurological scores of each rat were also performed at each time of intravenous administration. The neurological deficit score of each animal was evaluated according to the method described previously [33] . Briefly, forelimb and hindlimb flexion, forelimb motor function, postural reaction, and each animal's posture were observed. Each item was scored from 0–3 and the most severe animal scored 15 points. At day 15, animals were killed under sodium pentobarbital anaesthesia. Saline perfusion followed by brain removal was preformed, and six preselected coronal sections (from anterior 3.5 mm to anterior 13.5 mm), 2 mm in thickness, were made using a brain matrix (RBS-02, Neuroscience). For each section, haemorrhagic area was determined using computerized image analysis by Photoshop and Image J software. Generation of recombinant Cnm and application in mouse model Recombinant Cnm was generated as reported previously [34] . Briefly, the coding region for Cnm of strain TW871 was amplified by PCR, which was subcloned into the expression vectors pET-42a(+) (Novagen). Then, the resultant plasmids were transformed into Escherichia coli BL21 (DE3). The E. coli organisms were grown in Luria-Bertani broth containing kanamycin and tetracycline at 37 °C to the mid-exponential phase. Isopropylthio-β-d-galactoside (Wako Chemicals) was then added to give a final concentration of 1.0 mM, and the cultures were incubated for an extra 3 h to induce GST–Cnm protein synthesis. After that, the cells were collected and were suspended in 10 mM phosphate buffer, which was ultrasonicated on ice. Supernatants were obtained and purified using a glutathione Sepharose 4B column (GE Healthcare). The GST-fusion protein treated with PreScission Protease (GE Healthcare) at 4 °C was subjected to SDS–PAGE, and purified recombinant Cnm was obtained using GeBA flex-tube (Gene Bio Application). The collagen binding activity of recombinant Cnm protein was confirmed by the inhibition of TW295 adhesion to collagen layers ( Supplementary Fig. S5 ), and the dosages were determined as 10 and 100 μg according to the inhibition curve. Then, the recombinant Cnm protein was applied in mouse cerebral haemorrhage model as described above. Statistical analyses Statistical analyses were carried out with Prism 4 (GraphPad Software). Fisher's protected least significant difference, Student's t -tests, regression analysis and Bonferroni's method after analysis of variance (ANOVA) were performed. The results were considered significantly different when P <0.05. How to cite this article : Nakano, K. et al . The collagen-binding protein of Streptococcus mutans is involved in haemorrhagic stroke. Nat. Commun. 2:485 doi: 10.1038/ncomms1491 (2011).